Functional profiles of orphan membrane transporters in the life cycle of the malaria parasite Assigning function to orphan membrane transport proteins and prioritizing candidates for detailed biochemical characterization remain fundamental challenges and are particularly important for medically relevant pathogens, such as malaria parasites. Here we present a comprehensive genetic analysis of 35 orphan transport proteins of Plasmodium berghei during its life cycle in mice and Anopheles mosquitoes. Six genes, including four candidate aminophospholipid transporters, are refractory to gene deletion, indicative of essential functions. We generate and phenotypically characterize 29 mutant strains with deletions of individual transporter genes. Whereas seven genes appear to be dispensable under the experimental conditions tested, deletion of any of the 22 other genes leads to specific defects in life cycle progression in vivo and/or host transition. Our study provides growing support for a potential link between heavy metal homeostasis and host switching and reveals potential targets for rational design of new intervention strategies against malaria. Membrane transport proteins (MTP) transfer compounds across biological membranes and encompass diverse gene families, namely ion channels, ATP-dependent pumps and secondary active porters including those of the major facilitator superfamily. Together they play important physiological roles in, for example, nutrient uptake, disposal of waste products, shuttling of metabolites between organelles, and generation and maintenance of the electrochemical gradient. They critically determine safety and efficacy of drugs and are attractive therapeutic targets [1] . Accordingly, MTPs rank amongst the top five protein classes that are molecular targets of FDA-approved drugs [2] . Prominent examples in the WHO model list of essential medicines include ion channel blockers, for example, verapamil, and serotonin transporter (5-HTT) inhibitors, for example, fluoxetine [3] . In contrast to bacteria, archaea and fungi, parasitic protozoa such as Trypanosoma brucei and the malaria parasite Plasmodium falciparum allocate only a small proportion of their genomes (2–3%) to membrane transport ( Supplementary Fig. 1 ) [4] . P. falciparum encodes at least 122 MTPs [5] . Some MTPs play central roles during the pathogenic blood-stage proliferation of malaria parasites, for example, through the import of critical nutrients such as pantothenic acid [6] , [7] and isoleucine [8] , or mediate drug resistance, most notably against chloroquine through the chloroquine resistance transporter [9] , [10] . However, functions of the vast majority of Plasmodium transport proteins are inferred from homology to genes from model organisms [11] . For 39 gene products, functional or subcellular localization predictions remain elusive, rendering them orphan MTPs [5] . We reasoned that due to their phylogenetic distance to host MTPs they constitute particularly attractive targets for novel targeted malaria intervention approaches. A better and unbiased understanding of human and pathogen MTP gene function is central to pharmacogenomics and drug target validation [12] . Despite this research priority, few systematic experimental genetics studies of MTPs have been reported for any organism and merely in the context of genome-wide collections of gene deletion mutants in model organisms, such as Saccharomyces cerevisiae [13] , [14] . In the search for targets for novel prophylactic, therapeutic and transmission-blocking intervention strategies to fight malaria, we report here a broad characterization of the importance of orphan MTP orthologues during the complete life cycle of the murine malaria model parasite Plasmodium berghei by relatively fast and efficient experimental genetics approaches. Enrichment of putative flippases in vital gene candidates For three of the 39 P. falciparum orphan MTPs there is no rodent malaria parasite orthologue ( Fig. 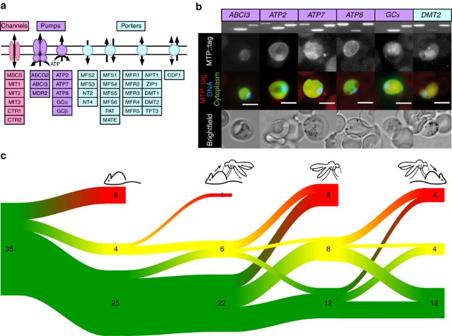Figure 1: Experimental genetics screen of malaria parasite orphan membrane transport proteins. (a) Schematic overview of the 35 conserved,P. bergheiorphan MTPs targeted in this study. (b) Endogenous fluorescent tagging of six MTPs refractory to targeted gene deletion to validate accessibility of gene loci. Diagnostic PCRs of the parental parasite populations (left, WT; centre, 5′ integration; right, 3′ integration; seeSupplementary Fig. 5for full gel pictures) and representative live fluorescent micrographs of blood-stage parasites are shown. Scale bars, 5 μm. (c) Sankey diagram for parasite development at four life cycle checkpoints. Parasite lines are enumerated and coloured according to complete arrest (red), slow development (<10% percentile; yellow), and normal growth (green). The Sankey diagram was created with the package riverplot (v. 0.5) available from CRAN (https://cran.r-project.org/web/packages/riverplot/). 1a ; Supplementary Table 1 ). In addition, GAP40 encodes a member of the glideosome motor complex [15] . As predicted, PbGAP40 is refractory to constitutive gene deletion ( Supplementary Fig. 2 ). Of the remaining 35 P. berghei orphan MTPs, only six (17%) were refractory to repeated gene deletion attempts, using two complementary strategies ( Fig. 2a,b ) [16] , [17] , strongly indicating essential roles during asexual blood-stage growth ( Figs 1b,c and 3 ). Corresponding gene deletion lines ( mtp − ) could not be generated, but we readily selected endogenously labelled mtp::tag lines ( Fig. 1b ). Live fluorescent imaging of intra-erythrocytic parasites revealed localization at the parasite–host interface (ATP2 and ATP8) or to intraparasitic structures and the surrounding membranes (ABCI3, ATP7, GCα and DMT2). Intriguingly, four essential genes encode signatures of aminophospholipid-transporting P 4 -type ATPases. These ATPases are restricted to eukaryotes and facilitate inward translocation of aminophospholipids thereby maintaining their asymmetrical enrichment at the membrane inner leaflet [18] . As lipid asymmetry is critical to normal cell functions, our data are consistent with a vital dependence of blood-stage malaria parasites on maintenance of lipid asymmetry. This potential vulnerability was previously unrecognized and might inform drug discovery programs. Figure 1: Experimental genetics screen of malaria parasite orphan membrane transport proteins. ( a ) Schematic overview of the 35 conserved, P. berghei orphan MTPs targeted in this study. ( b ) Endogenous fluorescent tagging of six MTPs refractory to targeted gene deletion to validate accessibility of gene loci. Diagnostic PCRs of the parental parasite populations (left, WT; centre, 5′ integration; right, 3′ integration; see Supplementary Fig. 5 for full gel pictures) and representative live fluorescent micrographs of blood-stage parasites are shown. Scale bars, 5 μm. ( c ) Sankey diagram for parasite development at four life cycle checkpoints. Parasite lines are enumerated and coloured according to complete arrest (red), slow development (<10% percentile; yellow), and normal growth (green). The Sankey diagram was created with the package riverplot (v. 0.5) available from CRAN ( https://cran.r-project.org/web/packages/riverplot/ ). 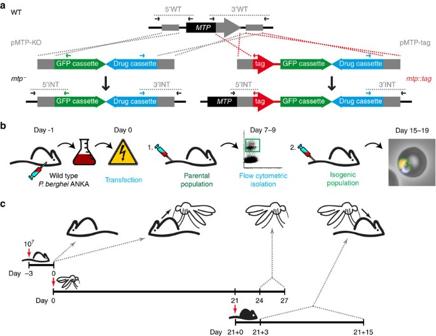Figure 2: Experimental genetics approaches employed to study 35 MTP. (a) Schematic representation of the generation ofmtp−andmtp::tagparasites. The 5′ and 3′ flanking regions of the target genes were cloned adjacent to the selection cassette resulting in the gene deletion transfection vector (pMTP-KO). For endogenous tagging, the carboxy terminus was cloned in frame with an mCherry-3xMyc tag and the 3′FR was cloned distal of the selection cassette, resulting in the endogenous tagging vector (pMTP-tag). By double crossover homologous recombination the targeted MTP was predicted to be either replaced or endogenously tagged with the fluorescent tag, respectively. (b) Schematic representation of theP. bergheitransfection protocol adapted from Matz and Kooij37. Cultured and synchronized schizonts are transfected and successfully modified parasites are selectedin vivousing pyrimethamine. When the parasitaemia is 0.1–1.0%, 50 isogenic mutant parasites are isolated by flow cytometry. (c) Schematic overview of the standardized phenotypic profiling protocol of four life cycle checkpoints looking at (1) blood-stage growth in the mouse, (2) exflagellation rates as a measure of mouse-to-mosquito transmission, (3) salivary gland sporozoite numbers, and (4) prepatency following infections by natural bites to follow mosquito-to-mouse transition and ability to complete the full life cycle. Full size image Figure 2: Experimental genetics approaches employed to study 35 MTP. ( a ) Schematic representation of the generation of mtp − and mtp::tag parasites. The 5′ and 3′ flanking regions of the target genes were cloned adjacent to the selection cassette resulting in the gene deletion transfection vector (pMTP-KO). For endogenous tagging, the carboxy terminus was cloned in frame with an mCherry-3xMyc tag and the 3′FR was cloned distal of the selection cassette, resulting in the endogenous tagging vector (pMTP-tag). By double crossover homologous recombination the targeted MTP was predicted to be either replaced or endogenously tagged with the fluorescent tag, respectively. ( b ) Schematic representation of the P. berghei transfection protocol adapted from Matz and Kooij [37] . Cultured and synchronized schizonts are transfected and successfully modified parasites are selected in vivo using pyrimethamine. When the parasitaemia is 0.1–1.0%, 50 isogenic mutant parasites are isolated by flow cytometry. ( c ) Schematic overview of the standardized phenotypic profiling protocol of four life cycle checkpoints looking at (1) blood-stage growth in the mouse, (2) exflagellation rates as a measure of mouse-to-mosquito transmission, (3) salivary gland sporozoite numbers, and (4) prepatency following infections by natural bites to follow mosquito-to-mouse transition and ability to complete the full life cycle. 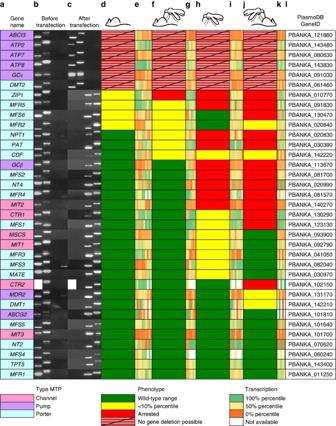Figure 3: Genetic screen of 35Plasmodium bergheimembrane transport proteins. The 6 essential and 29 targetable genes were clustered according to their phenotypes. For each gene the following information is provided: (a) gene name and MTP category colour-coded as indicated in the legend; (b) diagnostic PCR before transfection on DNA of WT parasites specific for 5′ and 3′ WT, 5′ and 3′ integration (note that for WTCTR2a single overarching PCR from 5′ to 3′ was performed; seeSupplementary Fig. 5for full gel pictures); (c) diagnostic PCR after transfection on DNA of parental transfected populations (6 essential genes) or isolated, isogenic mutant parasites (29 targetable genes) specific for 5′ and 3′ WT, 5′ and 3′ integration—absence of WT signals indicate 29 pure populations (seeSupplementary Fig. 5for full gel pictures); (d–k) alternating graphic representations of the phenotypes and transcription levels derived from refs38,39,40, colour coded as indicated in the legend; (d) blood-stage growth measured as pparasitaemia 3 days after infection of NMRI mice with 107parasites; (e) transcription percentiles ofP. bergheiring stages 4 hours post infection (h.p.i.; 2 ×), trophozoites 16 h.p.i. (2 ×), schizonts 22 h.p.i. (2 ×),P. yoeliischizonts (2 ×), and mixed blood stages (2 ×); (f) male gamete exflagellation levels three days after infection of NMRI mice with 107parasites; (g) transcription percentiles ofP. bergheigametocytes (2 ×) andP. yoeliigametocytes (4 ×); (h) number of salivary gland-associated sporozoites 21 days after blood meal; (i) transcription percentiles ofP. bergheiookinetes,P. yoeliimidgut-associated sporozoites 9 d.p.i. (2 × ), 10 d.p.i., salivary gland-associated sporozoites 14 d.p.i. (3 × ) and 15 d.p.i.; (j) prepatent period in two C57BL/6 mice following bites of 25 infectious mosquitoes (green, both mice became blood-film positive with an average prepatent period of ≤4.5 days; yellow, one mouse remained blood-film negative; red, both mice remained blood-film negative); (k) transcription percentiles ofP. yoeliiliver stages at 24, 36, 40 (2 × ) and 50 h.p.i.; (l) gene identification number. Full size image Figure 3: Genetic screen of 35 Plasmodium berghei membrane transport proteins. The 6 essential and 29 targetable genes were clustered according to their phenotypes. For each gene the following information is provided: ( a ) gene name and MTP category colour-coded as indicated in the legend; ( b ) diagnostic PCR before transfection on DNA of WT parasites specific for 5′ and 3′ WT, 5′ and 3′ integration (note that for WT CTR2 a single overarching PCR from 5′ to 3′ was performed; see Supplementary Fig. 5 for full gel pictures); ( c ) diagnostic PCR after transfection on DNA of parental transfected populations (6 essential genes) or isolated, isogenic mutant parasites (29 targetable genes) specific for 5′ and 3′ WT, 5′ and 3′ integration—absence of WT signals indicate 29 pure populations (see Supplementary Fig. 5 for full gel pictures); ( d – k ) alternating graphic representations of the phenotypes and transcription levels derived from refs 38 , 39 , 40 , colour coded as indicated in the legend; ( d ) blood-stage growth measured as pparasitaemia 3 days after infection of NMRI mice with 10 7 parasites; ( e ) transcription percentiles of P. berghei ring stages 4 hours post infection (h.p.i. ; 2 ×), trophozoites 16 h.p.i. (2 ×), schizonts 22 h.p.i. (2 ×), P. yoelii schizonts (2 ×), and mixed blood stages (2 ×); ( f ) male gamete exflagellation levels three days after infection of NMRI mice with 10 7 parasites; ( g ) transcription percentiles of P. berghei gametocytes (2 ×) and P. yoelii gametocytes (4 ×); ( h ) number of salivary gland-associated sporozoites 21 days after blood meal; ( i ) transcription percentiles of P. berghei ookinetes, P. yoelii midgut-associated sporozoites 9 d.p.i. (2 × ), 10 d.p.i., salivary gland-associated sporozoites 14 d.p.i. (3 × ) and 15 d.p.i. ; ( j ) prepatent period in two C57BL/6 mice following bites of 25 infectious mosquitoes (green, both mice became blood-film positive with an average prepatent period of ≤4.5 days; yellow, one mouse remained blood-film negative; red, both mice remained blood-film negative); ( k ) transcription percentiles of P. yoelii liver stages at 24, 36, 40 (2 × ) and 50 h.p.i. ; ( l ) gene identification number. Full size image Streamlined phenotyping of viable mtp − lines For 29 target genes (81%), transfection, selection and isolation of isogenic mtp – lines were successful ( Figs 1 , 2 , 3 ). We established a streamlined and standardized phenotypic screen ( Fig. 2c ), monitoring life cycle progression at four clearly defined checkpoints in the definitive host, female Anopheles mosquitoes, and the intermediate murine host. Following intravenous infection of outbred (NMRI) mice with 10 7 infected erythrocytes, parasitaemia (i) and male gamete exflagellation (ii) were quantified three days later. Anopheles stephensi mosquitoes were allowed to feed on these mice and salivary gland-associated sporozoites (iii) were enumerated at least three weeks later. Natural transmission (iv) was monitored after exposure of C57BL/6 mice to 25 mtp − -infected mosquitoes. This screen identified only seven gene deletions with no apparent deficiency at any checkpoint, indicative of dispensable and/or redundant roles for parasite propagation and host switch ( Figs 1c and 3 ; Supplementary Table 2 ). Ablation of nine MTP genes resulted in defects at a single stage or at multiple checkpoints. Despite the observed deficiencies, these mtp − lines completed the life cycle, illustrating that life cycle bottlenecks can be readily compensated by subsequent propagation phases in partly attenuated parasites. A selection of seven mutants exemplified how such an initial defect does not need to preclude subsequent normal development. Sporozoite numbers for the mfs6 − and mfr2 − strains are within the wild-type (WT) range despite severely reduced exflagellation rates, while five mutant lines that show reduced sporozoite numbers transmit normally. The remaining thirteen mtp − lines (36%) demonstrated a complete life cycle arrest abrogating transmission between mice. Defects during asexual or sexual blood-stage development We next determined the parasite multiplication rates (PMR) of the four parasite lines that showed the lowest mean parasitaemias in the phenotyping screen ( Fig. 4a ). Thus, we could rule out a growth defect for mfr2 − but uncovered replication defects for zip1 − (68% PMR), mfs6 − (55% PMR) and mfr5 − (36% PMR) parasites, resulting in swift out-competition by WT parasites. Growing at a third of the rate of WT blood-stage parasites, MFR5 -deficient parasites are the slowest replicating mutants isolated to date and we independently confirmed this outcome ( Supplementary Fig. 3 ). 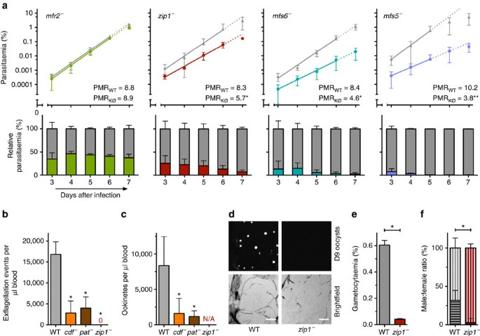Figure 4: Blood infection and mouse-to-mosquito transition of selectedmtp−parasites. (a) Blood infection of the four slowest growingmtp−parasite lines (mfr2−,zip1−,mfs6−, andmfr5−) in competition with WT (grey). Shown are mean parasitaemias±s.d. from at least three experiments (top) and the kinetics of relative parasite distribution (bottom) from day 3 to 7 after injection. **P<0.01; *P<0.05 (two-tailed F-test). (b) Male gamete exflagellation and (c)in vitroookinete formation for selectedmtp−(cdf−,pat−andzip1−) parasite lines. Shown are mean values±s.d. *P<0.05 (Mann–Whitney test). (d) Oocysts formation is abrogated inzip1−parasites. Bars, 100 μm. (e) Gametocyte conversion is defective inzip1−parasites. Shown are mean values±s.d. *P<0.05 (Mann–Whitney test). (f) Ratio of male (bottom, horizontal lines) and female (top, vertical lines) gametocytes of the total formed in WT andzip1−infections shows that male gametocyte formation inzip1−parasites is more defective than female gametocyte formation. Shown are mean values±s.d. *P<0.05 (Mann–Whitney test). Figure 4: Blood infection and mouse-to-mosquito transition of selected mtp − parasites. ( a ) Blood infection of the four slowest growing mtp − parasite lines ( mfr2 − , zip1 − , mfs6 − , and mfr5 − ) in competition with WT (grey). Shown are mean parasitaemias±s.d. from at least three experiments (top) and the kinetics of relative parasite distribution (bottom) from day 3 to 7 after injection. ** P <0.01; * P <0.05 (two-tailed F-test). ( b ) Male gamete exflagellation and ( c ) in vitro ookinete formation for selected mtp − ( cdf − , pat − and zip1 − ) parasite lines. Shown are mean values±s.d. * P <0.05 (Mann–Whitney test). ( d ) Oocysts formation is abrogated in zip1 − parasites. Bars, 100 μm. ( e ) Gametocyte conversion is defective in zip1 − parasites. Shown are mean values±s.d. * P <0.05 (Mann–Whitney test). ( f ) Ratio of male (bottom, horizontal lines) and female (top, vertical lines) gametocytes of the total formed in WT and zip1 − infections shows that male gametocyte formation in zip1 − parasites is more defective than female gametocyte formation. Shown are mean values±s.d. * P <0.05 (Mann–Whitney test). Full size image We detected substantial reductions in male gamete exflagellation and ookinete formation for pat − and cdf − ( Fig. 4b,c ). As cdf − , but not pat − , parasites were capable of completing transmission ( Fig. 3 ; Supplementary Table 2 ) PAT likely exerts additional roles following ookinete formation. Remarkably, zip1 − was the only mutant that completely failed to form flagella and, thus, ookinetes and oocysts ( Fig. 4b–d ). In this mutant, gametocyte numbers were reduced by 80% ( Fig. 4e ) but most strikingly the male:female ratio was strongly skewed towards female production ( Fig. 4f ). CDF and ZIP1 might participate in the transport of heavy metal ions [5] , [19] . Our phenotyping, and the known role of a copper-transporting P 1B1 -type ATPase (CuTP) in gamete fertility [20] , underscore a possible central role for heavy metal homeostasis in malaria parasites fertility and, perhaps, the germ line of other eukaryotes. Defects during mosquito-stage development Over one third of the targeted MTP genes displayed a first defect in sporozoite colonization of the salivary glands ( Figs 1c and 3 , and Supplementary Table 2 ). These included four of six predicted channels ( CTR1 , MIT1 , MIT2 and MSCS ), highlighting their importance for the extracellular growth stage of the parasite. Five mtp − lines did not produce any salivary gland-associated sporozoites and two mutants failed to transmit following strongly reduced sporozoite production. In-depth phenotyping of three representative mutants ( ctr1 − , nt4 − and mfr4 − ) showed normal midgut colonization but attenuation of oocyst development, resulting in either no sporozoites ( mfr4 − ) or severely reduced sporozoite colonization of salivary glands ( ctr1 − and nt4 − ; Fig. 5 ). 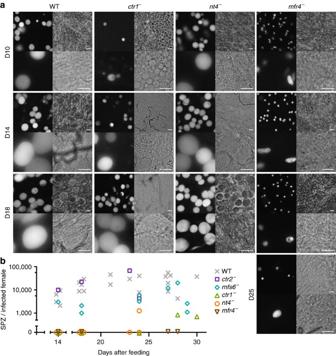Figure 5: Critical roles for selectedMTPsin sporogony. (a) Mosquito midguts were isolated at 10, 14, 18 and 25 (mfr4−only) days after the infectious blood meal. Shown are representative live micrographs of the highly expressed cytoplasmic GFP (left panels) and bright field images (right panels) recorded with 40 × (top panels) and 100 × (bottom panels) objectives. Note the elongated ookinete-like shape rather than a round and spherical appearance of themfr4−oocysts in the higher magnification. Scale bars, 20 μm. (b) Enumeration of sporogony in five recombinant parasite lines. Midgut-associated sporozoites were isolated and quantified on day 14 after the blood meal. Salivary gland-associated sporozoite numbers were determined over the course of two weeks starting on day 18 after the infectious blood meal. Data combined from at least three independent feeding experiments. Figure 5: Critical roles for selected MTPs in sporogony. ( a ) Mosquito midguts were isolated at 10, 14, 18 and 25 ( mfr4 − only) days after the infectious blood meal. Shown are representative live micrographs of the highly expressed cytoplasmic GFP (left panels) and bright field images (right panels) recorded with 40 × (top panels) and 100 × (bottom panels) objectives. Note the elongated ookinete-like shape rather than a round and spherical appearance of the mfr4 − oocysts in the higher magnification. Scale bars, 20 μm. ( b ) Enumeration of sporogony in five recombinant parasite lines. Midgut-associated sporozoites were isolated and quantified on day 14 after the blood meal. Salivary gland-associated sporozoite numbers were determined over the course of two weeks starting on day 18 after the infectious blood meal. Data combined from at least three independent feeding experiments. Full size image Defects during liver-stage development Only two mutants with normal sporozoite production, ctr2 − and mfs6 − , had a distinct defect during natural transmission ( Figs 3 and 5b ; Supplementary Table 2 ). The observed defect in natural transmission of ctr2 − parasites ( Fig. 6a ) was alleviated by intravenous, but not subcutaneous, syringe delivery of sporozoites ( Fig. 6b ), and was largely independent of gliding motility ( Fig. 6c ) or liver-stage maturation ( Fig. 6d,g ). These findings indicate an important role for CTR2 in sporozoite transmission in vivo . The critical roles of an alternative zinc–iron permease ( ZIPCO ) during liver-stage development [21] , and of CTR1 and CTR2 described herein, support a link between heavy metal homeostasis and parasite–host switch. Furthermore, iron deprivation via hepcidin inhibits liver-stage growth [22] . Taken together, the growing evidence indicates that heavy metal homeostasis might become a useful molecular target for causal prophylactic strategies. 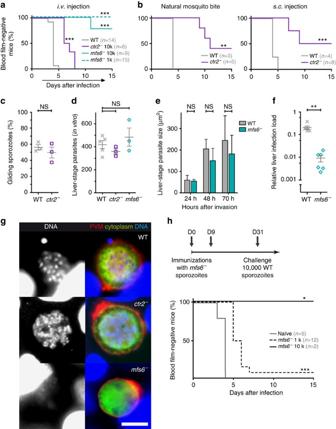Figure 6: Defective transmission and liver-stage maturation inctr2−andmfs6−parasites. (a) Kaplan–Meier analysis of infection by intravenous injection of 10,000 (WTn=14,ctr2−n=6,mfs6−n=9) or 1,000 (mfs6−n=15) salivary gland-associated sporozoites. ***P<0.001 (Log-rank Mantel–Cox). (b) Kaplan–Meier analysis of infection by exposure to infected mosquitoes (left; WTn=3,ctr2−n=5) and subcutaneous injection of 10,000 isolated salivary gland-associated sporozoites (right; WTn=4,ctr2−n=8). ***P<0.001; **P<0.01 (Log-rank Mantel–Cox). (c) Gliding motility ofctr2−sporozoites (NS, non-significant; Mann–Whitney test). (d) Numbers of maturectr2−andmfs6−liver stages in cultured hepatoma cells (NS, non-significant; Kruskal–Wallis with Dunn’s post test). (e) Surface areas of developingmfs6−liver-stage parasites. Shown are mean values±s.d. (NS, non-significant; Mann–Whitney test). (f) Parasite liver load in WT- andmfs6−-infected C57BL/6 mice. **P<0.01 (two-tailed Mann–Whitney). (g) Aberrant liver-stage maturation ofmfs6−parasites. Shown are immunofluorescent micrographs of mature liver-stage-infected hepatoma cells. (UIS4, red; HSP70, green; Hoechst, blue). Scale bar, 10 μm. (h) Immunization/challenge protocol (top) for vaccination with genetically arrestedmfs6−sporozoites. Kaplan–Meier analysis (bottom) of blood infection after sporozoite challenge infection inmfs6−-immunized mice. ***P<0.001; *P<0.05 (Log-rank Mantel–Cox). Figure 6: Defective transmission and liver-stage maturation in ctr2 − and mfs6 − parasites. ( a ) Kaplan–Meier analysis of infection by intravenous injection of 10,000 (WT n =14, ctr2 − n =6, mfs6 − n =9) or 1,000 ( mfs6 − n =15) salivary gland-associated sporozoites. *** P <0.001 (Log-rank Mantel–Cox). ( b ) Kaplan–Meier analysis of infection by exposure to infected mosquitoes (left; WT n =3, ctr2 − n =5) and subcutaneous injection of 10,000 isolated salivary gland-associated sporozoites (right; WT n =4, ctr2 − n =8). *** P <0.001; ** P <0.01 (Log-rank Mantel–Cox). ( c ) Gliding motility of ctr2 − sporozoites (NS, non-significant; Mann–Whitney test). ( d ) Numbers of mature ctr2 − and mfs6 − liver stages in cultured hepatoma cells (NS, non-significant; Kruskal–Wallis with Dunn’s post test). ( e ) Surface areas of developing mfs6 − liver-stage parasites. Shown are mean values±s.d. (NS, non-significant; Mann–Whitney test). ( f ) Parasite liver load in WT- and mfs6 − -infected C57BL/6 mice. ** P <0.01 (two-tailed Mann–Whitney). ( g ) Aberrant liver-stage maturation of mfs6 − parasites. Shown are immunofluorescent micrographs of mature liver-stage-infected hepatoma cells. (UIS4, red; HSP70, green; Hoechst, blue). Scale bar, 10 μm. ( h ) Immunization/challenge protocol (top) for vaccination with genetically arrested mfs6 − sporozoites. Kaplan–Meier analysis (bottom) of blood infection after sporozoite challenge infection in mfs6 − -immunized mice. *** P <0.001; * P <0.05 (Log-rank Mantel–Cox). Full size image Genetically modified Plasmodium parasites that are unable to undergo liver-to-blood-stage conversion can be used to experimentally immunize mice resulting in sterile protection against future sporozoite challenge infections [23] . Broadly, these genetically arrested parasites fall into two distinct classes: (1) early arrested liver stages that fail to grow in cultured hepatoma cells and show a reduced liver load in vivo , and (2) late arrested parasites that initially grow normally but have a defect in liver-stage merozoite formation, correlating with a high liver load in infected mice. Only one of the mutant strains, mfs6 − , fulfilled criteria for testing in a preclinical immunization/challenge protocol as a genetically arrested parasite vaccine. Fine analysis of the observed defect of mfs6 − parasites in natural transmission revealed occasional (2 out of 9) delayed breakthrough blood infections only after high-dose inoculations with 10,000 mfs6 − sporozoites ( Fig. 6a ). Numbers and sizes of liver-stage parasites in cultured hepatoma cells were not different from WT parasites ( Fig. 6d,e ), though a trend towards slightly reduced sizes in maturing stages was observed. Furthermore, we did not detect liver-stage merozoites in mfs6 − -infected cell cultures. In contrast with late arresting liver-stage mutants, mfs6 − liver load was largely reduced in vivo ( Fig. 6f ). Intriguingly, DNA staining revealed distorted nuclei displaying weak signals only ( Fig. 6g ; Supplementary Fig. 4 ), lending support to an apparent replication deficit. Therefore, infections with mfs6 − parasites display defining signatures of late arrest (numbers and morphology) and early arrest (DNA content). Immunizations with late arrested parasites elicit particularly potent and lasting protection [24] , [25] . To test the vaccine potential of mfs6 − parasites, we immunized C57BL/6 mice with two low doses of 1,000 mfs6 − sporozoites. The immunized mice displayed an average delay to blood infection of 1–2 days upon high-dose sporozoite challenge and one mouse was sterily protected from re-infection ( Fig. 6h ). Despite this promising result, additional bioengineering efforts, including generation of multiple gene deletions, are required before a late arresting genetically attenuated whole-parasite vaccine can be translated to P. falciparum parasites and potential clinical trials. Concluding remarks Classical reverse genetics and post-genomic approaches continue to provide increasing insights in the functioning of membrane transport proteins in the model yeast S. cerevisiae [26] . In the present study, we have presented a relatively rapid experimental system to uncover phenotypes and assign in vivo functions to a significant proportion (30%) of the Plasmodium transporters, which could not be inferred on the basis of motifs and sequence similarities with established unicellular model organisms. Such insights contribute to a better understanding of Plasmodium metabolism and host cell adaptation, which forms the basis for the rational development of innovative malaria intervention strategies. Our data show that MTPs, with the notable exception of ATP-dependent pumps, play a less prominent role than anticipated. Systematic target validation is a critical component of the anti-malarial drug and vaccine discovery process. This is exemplified herein by the prophylactic and transmission-blocking potential of targeting an MTP putatively involved in heavy metal homeostasis during malaria parasite–host switches; the vaccine potential of genetically arrested parasites that lack a parasite-specific MTP of the major facilitator superfamily; and the possibility for therapeutic intervention targeting putative aminophospholipid translocases. Experimental animals All animal work was conducted in accordance with the German ‘Tierschutzgesetz in der Fassung vom 18. Mai 2006 (BGBl. I S. 1207)’, which implements the directive 86/609/EEC from the European Union and the European Convention for the protection of vertebrate animals used for experimental and other scientific purposes. The protocol was approved by the ethics committee of MPI-IB and the Berlin state authorities (LAGeSo Reg# G0469/09). We used 6-to-8 weeks old female mice from Charles River: C57BL/6 mice for sporozoite infections and NMRI mice for all other parasite infections. Generation of mtp − and mtp::tag parasites All recombinant parasite lines were generated in the P. berghei strain ANKA reference line cl15cy1 (ref. 27 ) through a gene replacement strategy via double crossover/ends-out homologous recombination ( Fig. 2a ). All sequences of the oligonucleotides with the restriction sites and approximate sizes can be found in Supplementary Table 3 . Fragments of 400–650 bp in the 3′ flanking regions of the genes of interest were amplified by using the 3′ fragment forward and reverse primer combinations (3′MTP-F-AvrII and 3′MTP-R-KpnI). The 3′ fragments were cloned using the indicated restriction sites into the pBAT-SIL6 vector [28] , resulting in intermediate vectors (pMTP-IM). For completion of the gene deletion vectors (pMTP-KO), 400–650 bp fragments in the 5′ flanking regions of the target genes were amplified using the 5′ fragment forward and reverse primer combinations (5′MTP-F-SacII and 5′MTP-R-HpaI) and cloned into the pMTP-IM vectors from which the mCherry-3xMyc tag sequence was removed by restriction digestion with SacII and PvuII. For completion of the tagging vectors (pMTP-tag), 400–650 bp fragments at the carboxy-terminal (CT) ends of the coding sequences were amplified using the CT fragment forward and reverse primer combinations (CT-MTP-F-SacII and CT-MTP-R-HpaI) and cloned into the pMTP-IM vectors using SacII and HpaI resulting in in-frame fusions of the CT coding regions with the mCherry-3xMyc tag. All transfection plasmids were verified by commercial Sanger sequencing and linearized with the enzymes ScaI and SalI. We transfected P. berghei strain ANKA with 5 μg linearized transfection plasmid DNA using standard procedures ( Fig. 2b ) [27] . In brief, blood of a mouse infected with WT parasites is harvested by cardiac puncture and cultured overnight. Following maturation, the parasites fail to egress and arrest at the schizont stage. These schizonts are purified and transfected with the targeting constructs. Transfected merozoites are injected intravenously into a naïve mouse. Administration of pyrimethamine in the drinking water favours the growth of successfully modified parasites, which now also express a fluorescent protein. When the parasitaemia is 0.1–1.0% (typically 7–9 days after transfection), 50 mutant parasites are isolated by flow cytometry and transferred to a naïve mouse [17] . Eight to ten days after injection, the isogenic parasite line can be harvested, stored or transferred and tested. When three repeated gene deletion attempts were unsuccessful, refractoriness of the genes was confirmed using the available, corresponding Plasmo GEM vectors ( GAP40 , PbG01-2401a08; ABCI3 , PbG01-2370b05; ATP2 , PbG01-2339e11; GCα , PbG01-2474g01) [16] . These independent transfection vectors harbour significantly longer homology arms and integrate more efficiently providing a further, more stringent test for essentiality. Accessibility of the locus for genetic manipulation was confirmed using the pMTP-tag vectors. Correct integration of the transfection vectors in the isogenic parasite lines and absence of contaminating WT parasites was verified by genotyping PCR ( Figs 2a and 3 ; Supplementary Table 3 ). In general, for each target gene two primer combinations for genotyping purposes were designed just outside the regions used for homologous recombination, one flanking the 5′ fragment (5′MTP-F and 5′MTP-R) and one spanning both the CT- and 3′ fragments (3′MTP-F and 3′MTP-R). To confirm the predicted integration events, the gene-specific primers were combined with generic pBAT-SIL6-specific primers (5′HSP70rev for 5′ integration in mtp − lines, mCherryRev for 5′ integration in mtp::tag lines, and 5′DHFRrev for 3′ integration in both). Standardized phenotyping screen To facilitate a comprehensive phenotypic profiling of the large number of recombinant mtp − parasite lines, we standardized our life cycle progression analysis to maximize functional read-outs over invested time and resources, particularly with regard to the number of experimental animals required. Figure 2c provides a schematic of this protocol, which starts with the intravenous injection of 10 7 blood-stage parasites into naïve NMRI mice. Three days later, blood-stage parasitaemia was counted by microscopic examination of Giemsa-stained thin blood films and male gamete exflagellation rates were determined as described below. For transmission, 25 female naïve A. stephensi Sind-Kasur strain mosquitoes [29] were placed into a single cup, starved for at least 8 h, and fed on a mtp − -infected mouse for 30 min. After 21 days, infected mosquitoes were starved for at least 8 h and fed on naïve C57BL/6 mice. From 3 to 15 days after the infectious mosquito bites, blood-stage infection was monitored by microscopic examination of Giemsa-stained thin blood films. At 24–27 days after the mosquito blood meal, salivary gland-associated sporozoites were isolated and quantified. Blood-stage development and live fluorescence imaging Blood-stage development of selected mtp − lines was analysed using a flow cytometry-based intravital competition assay, growing recombinant parasite lines in competition with a strongly fluorescent reference strain (Beryellow or Berred) within a single mouse [30] . Data from the exponential growth phase, that is, with parasitaemia <1%, fitted a linear regression well ( r 2 ≥0.99) and allowed the calculation of the PMR from the slopes. For live protein localization, a drop of tail blood from an infected mouse was mixed with 200 μl pre-warmed RPMI 1640 complemented with 0.2 μl of the DNA-dye Hoechst 33342 (Invitrogen) and distributed onto poly- L -lysine coated cover slips. Cells were allowed to settle for 5 min at 37 °C. Next, cover slips were washed three times with pre-warmed RPMI, inverted and sealed. Images were recorded on a Zeiss AxioObserver Z1 epifluorescence microscope, equipped with a Zeiss AxioCam MRm camera, and processed minimally with Fiji [31] . Sexual blood-stage development and ookinete cultures Detailed analyses of sexual development was largely performed as described [20] . Mice were infected with 10 7 blood-stage parasites. After 3 days, gametocyte conversion rates and male:female gametocyte ratios were determined by microscopic examination of Giemsa-stained thin blood films. For exflagellation analysis, 5 μl of tail blood was mixed immediately with 125 μl RPMI 1640 complemented with 50 μM xanthurenic acid, that was pre-warmed at 20 °C. Immediately, 10 μl cell suspension was transferred into a Neubauer chamber and incubated at 20 °C. Exflagellation centres were quantified by microscopic observation at 400 × magnification from 12 to 18 min. Finally, mice were bled by heart puncture and 1 ml blood was transferred immediately into a small cell culture flask containing 10 ml complete ookinete medium (RPMI 1640 with L -glutamine and 25 mM HEPES supplemented with 100 mM sodium bicarbonate, 125 U ml −1 penicillin/streptomycin, 10% fetal calf serum and 50 μM xanthurenic acid, pH 8.0). After 18–24 h incubation at 20 °C and 80% humidity, the ookinete culture was centrifuged in a 50 ml reaction tube for 8 min at 1,800 r.p.m. (560 g ) without brake. The pellet was resuspended with freshly prepared cold 0.17 M ammonium chloride solution and incubated for 10–15 min on ice. Ookinetes were collected by centrifugation at 4 °C and 2,100 r.p.m. (760 g ) for 15 min. The pellet was transferred into a 2 ml reaction tube and washed twice with PBS. The enriched ookinete suspension was then diluted appropriately, 10 μl of it transferred into a Neubauer chamber and quantified by microscopic examination at 400 × magnification. Mosquito-stage development and live fluorescence imaging A. stephensi mosquitoes were raised in a 14 h light/10 h dark cycle at 75% humidity using standard techniques [32] . Uninfected and infected mosquitoes were kept at 28 and 20 °C, respectively. Midgut sporozoites were isolated and quantified 14 days after the mosquito blood meal. Salivary gland-associated sporozoites were isolated and quantified between day 18 and 30 following the start of the mosquito infection. To visualize mosquito-stage development, midguts were isolated in RPMI 1640 supplemented with 2% BSA at 10, 14, 18 and 25 days after the mosquito blood meal. Mosquito midguts were placed on a glass slide and images recorded immediately using a Leica DMR epifluorescence microscope with 40 × and 100 × objectives. Gliding motility assay Glass slides with distinct wells were coated with 3% BSA in RPMI at 37 °C for 20 min. Overall 10,000 sporozoites in RPMI/3% BSA were added onto each well. Samples were placed at 37 °C in a humid chamber to allow sporozoites to settle and glide for 45 min. The parasites were fixed with 4% PFA for 15 min. Parasites and their trails were stained with anti-CSP antiserum (1:500 dilution—kindly provided by K. Müller, MPI-IB, Berlin). Primary antibodies were detected by fluorescently labelled secondary goat anti-mouse IgG Alexa Fluor 488 conjugated antibodies (1:1,000 dilution, Invitrogen). Sporozoites with trails that extended longer than one circle were scored as gliding. Data were obtained in three independent assays using salivary gland-associated sporozoites isolated from mosquitoes that were fed simultaneously. Transmissions to mice and quantification of liver loads For natural transmission, infected mosquitoes were starved for at least 8 h before feeding on anesthetized naïve C57BL/6 mice. For intravenous and subcutaneous injections in C57BL/6 mice, the desired numbers of sporozoites, typically 10,000, were isolated from infected mosquito salivary glands and injected in a volume of 100 μl into the tail vein or a skin fold on the back. To quantify the relative parasite liver infection load, 10,000 sporozoites were injected intravenously into C57BL/6 mice. After 44 h, the mice were sacrificed, RNA was isolated from infected livers, and transcribed into cDNA as described previously [33] . Quantitative real time PCR was performed on WT and mutant cDNA by using primers specific for P. berghei 18S rRNA and mouse glyceraldehyde-3-phosphate dehydrogenase ( GAPDH ) [33] . The mRNA level of P. berghei 18S rRNA was calculated relative to the mouse GAPDH levels. In vitro liver-stage growth and immunofluorescence imaging To study liver-stage development, in vitro cultured human hepatoma (Huh7) cells [34] were infected with 10,000 sporozoites using standard techniques as described previously [25] . After 24, 48 or 70 h, liver-stage parasites were fixed and permeabilized with ice-cold methanol and stained with the DNA-dye Hoechst 33342 (Invitrogen), rabbit anti-UIS4 antibodies (1:500 dilution [35] ), and mouse anti-HSP70 antibodies (1:300 dilution [36] ). Primary antibodies were detected by fluorescently labelled goat anti-mouse/rabbit IgG Alexa Fluor 488/546 conjugated antibodies (1:1,000 dilution, Invitrogen). Liver-stage parasites were counted and images recorded on a Zeiss AxioObserver Z1 epifluorescence microscope, equipped with a Zeiss AxioCam MRm camera, and processed minimally with Fiji [31] . Immunizations with mfs6 − sporozoites C57BL/6 mice were immunized with two doses of 1,000 or 10,000 mfs6 − sporozoites by intravenous injection at a 9-day interval. Mice that remained parasite-free were challenged three weeks after the final immunization with 10,000 WT sporozoites. Blood-stage infection was monitored daily from days 3–15 after infection by microscopic examination of Giemsa-stained thin blood films. How to cite this article: Kenthirapalan, S. et al . Functional profiles of orphan membrane transporters in the life cycle of the malaria parasite. Nat. Commun. 7:10519 doi: 10.1038/ncomms10519 (2016).